Source time function properties indicate a strain drop independent of earthquake depth and magnitude The movement of tectonic plates leads to strain build-up in the Earth, which can be released during earthquakes when one side of a seismic fault suddenly slips with respect to the other. The amount of seismic strain release (or ‘strain drop’) is thus a direct measurement of a basic earthquake property, that is, the ratio of seismic slip over the dimension of the ruptured fault. Here the analysis of a new global catalogue, containing ~1,700 earthquakes with magnitude larger than 6, suggests that strain drop is independent of earthquake depth and magnitude. This invariance implies that deep earthquakes are even more similar to their shallow counterparts than previously thought, a puzzling finding as shallow and deep earthquakes are believed to originate from different physical mechanisms. More practically, this property contributes to our ability to predict the damaging waves generated by future earthquakes. Earthquakes occur over a broad range of magnitudes, from microearthquakes with negative magnitudes to giant subduction earthquakes with magnitudes around 9 (for example, 2004 Sumatra earthquake and 2011 Tohoku-Oki earthquake). In terms of seismic moment, which is proportional to the product of the seismic fault area and average slip, the earthquake size spans over >15 orders of magnitude. Does the earthquake mechanism remain similar despite this extreme variability of sizes? This question has motivated the pioneering works of Aki [1] and Kanamori and Anderson [2] , and these studies indicated that shallow earthquakes tend to release a similar amount of shear stress (0.1–10 MPa), independent of their magnitude. The constant stress drop hypothesis has since been confirmed, using a larger number of earthquakes [3] and over a wider magnitude range [4] . On the other hand, deep earthquakes (50–670 km) have been globally shown to have a higher stress drop (typically one order of magnitude [5] , [6] ), but the more detailed features of the stress drop depth evolution have remained unclear [7] , [8] , [9] , [10] , [11] . The stress drop Δ σ is simply expressed by Δ σ=K μS/L , where μ, S, L and K are the Earth rigidity, the average slip, a characteristic rupture dimension and a coefficient close to 1 (ref. 2 ), respectively. In a bidimensional source model (for example, elliptical), the stress drop can be written as: where M 0 is the seismic moment. As the characteristic rupture dimension is difficult to evaluate for the majority of earthquakes, most studies determine it indirectly through estimations of temporal or spectral seismogram values, assuming a constant rupture velocity. Both temporal and spectral approaches require an appropriate modelling of the seismic propagation effects to isolate the seismic source contribution. Spectral methods are based on the determination of the corner frequency of the seismograms [3] , [12] , [13] , [14] assuming a particular rupture model. The determination of the corner frequency is not straightforward, as it depends on the spectral fall-off rate and can be made uncertain by the smoothness of the transition between low- and high-frequency regimes [15] . Temporal methods generally use the duration T of the source time function (STF), obtained after deconvolution of the Green’s function from the seismograms [11] , [16] , [17] . The STF represents the seismic moment rate as a function of time and T is therefore an objective measurement of the earthquake duration. T is directly related to the source dimension L through rupture velocity, and assuming that the rupture velocity itself is proportional to the shear velocity V S , we have: Several studies [5] , [18] support this hypothesis, although they tend to indicate that the average rupture velocity for deep earthquakes is about 0.6 V S , somewhat slower than the 0.7–0.8 V S empirically determined for shallow earthquakes [16] , [19] . Given this small difference, the limited number of deep earthquakes for which rupture velocity can be accurately determined, and a known tendency of underestimating the rupture velocity of deep earthquakes [20] , no systematic trend of the rupture velocity is considered in most of this study. The effects of such a depth dependency of the rupture velocity will be addressed at the end of the results section. Using equations (1) and (2), we expect: The practical determination of T may suffer from subjective criteria to determine when the STFs actually begins and ends. Moreover, in the case that an earthquake is composed of two (or more) slip patches separated in time, the stress drop derived from the earthquake duration is underestimated. That is why it is useful to also measure the peak value of the STF (maximum moment rate) F m . As M 0 T F m (seismic moment is the temporal integral of the STF), F m evolves as: The dependence of the STF amplitude, less known than the dependence of the STF duration, was already pointed out by Houston [17] . Equations (3) and (4) can also be written in terms of strain drop Δ ε , simply proportional to S/L, and Earth density ρ : A recently developed method, called SCARDEC [21] , provides simultaneous access to the focal mechanism, seismic moment, depth and STFs of all earthquakes with moment magnitude M w >6. As SCARDEC is fully automated [22] , we can easily obtain the STFs for an unprecedented number of earthquakes, spanning the whole depth range from Earth’s surface to ~660 km depth. Past studies using STFs were restricted to deep earthquakes [7] , [8] , [11] , [23] or to a limited STF catalogue [9] , [16] , [17] , [24] , [25] . Here we show, via analysis of the exhaustive SCARDEC STF database (1,700 earthquakes), that shallow earthquakes (depth <50 km, 1,200 events) have individual variations of their stress drops, but the general trend confirms that the constant stress drop hypothesis is well respected. Deeper earthquakes have a larger stress drop, but this depth evolution is shown to be well explained by the rigidity increase in the Earth, implying that the strain drop remains constant. In other words, it indicates that, independent of the earthquake depth, magnitude 6 and larger earthquakes keep on average a similar ratio between seismic slip and dimension of the main slip patch. 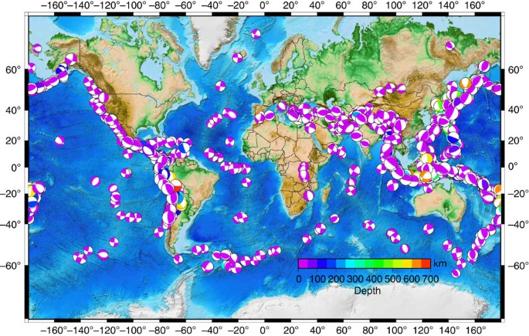Figure 1: Geographical distribution of the 1,700 earthquakes. STF was extracted for each of the 1,700 earthquakes shown on the map. Focal mechanisms are shown by the classical ‘beach ball’ representation, and depth is indicated by the colour scale. The size of a beach ball is proportional to the magnitude (Mw), ranging fromMw=6 earthquakes to the 2011Mw=9.1 Tohoku-Oki earthquake (Japan). SCARDEC STFs Figure 1 shows the locations and focal mechanisms of ~1,700 earthquakes for which a reliable STF has been extracted. Supplementary Figs S1–S3 show that first-order source parameters (seismic moment, depth and moment tensor) are found consistent with the Global Centroid Moment Tensor (GCMT) reference method [26] , [27] . This implies that STF characteristics can be safely compared with the SCARDEC depth and magnitude estimates without biasing the results, which is self-consistent compared with relying on external information. Compared with a past global STF catalogue developed by Ruff and colleagues [24] , SCARDEC catalogue has the advantages of containing many more events and of modelling more accurately large-magnitude earthquakes (above magnitude 7–7.5). Figure 1: Geographical distribution of the 1,700 earthquakes. STF was extracted for each of the 1,700 earthquakes shown on the map. Focal mechanisms are shown by the classical ‘beach ball’ representation, and depth is indicated by the colour scale. The size of a beach ball is proportional to the magnitude ( M w ), ranging from M w =6 earthquakes to the 2011 M w =9.1 Tohoku-Oki earthquake (Japan). Full size image For each of these earthquakes, the STF duration T and its peak moment rate F m have been measured, as shown in Fig. 2 , for several representative cases. 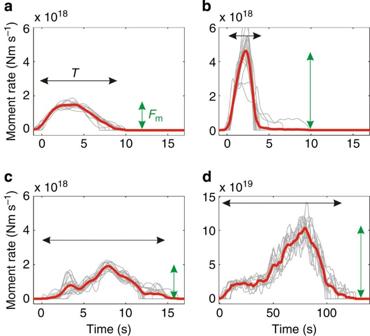Figure 2: Determining the characteristics of the STFs. In all subfigures, the STFs extracted from P waves recorded at individual seismic stations are shown in light grey and their averages are shown in thick red. The durationTof the average STF is indicated by the black arrow and the peak valueFmis shown by the green arrow. The end of the rupture (required to determineT) is defined here by the last point where the average STF is larger than 0.1Fm. Panelsa–cdemonstrate threeMw=6.6 earthquakes, occurring in Chile (14 July 2010, depth=23 km), Indonesia (11 November 2008, depth=107 km) and Papua New Guinea (11 December 2005, depth=9 km), respectively. These three cases are displayed with the same horizontal and vertical scales to illustrate the differences. The Chile earthquake (a) is a classical shallow earthquake, with a simple smooth STF.TandFmare on the order of 9 s and 1.6 1018Nm s−1, respectively. The Indonesia earthquake (b) is also simple, but like most deep earthquakes, its durationT(3–4 s) is shorter and its peak valueFm(4.7 1018Nm s−1) is larger. The Papua New Guinea earthquake (c) illustrates the case of a more complex STF, where several subevents are present and where the determination of the end of the rupture is dependent on subjective criteria. The total durationTis then more uncertain, and its meaning is more difficult to interpret. On the other hand,Fmcan still be objectively measured and can be related to the characteristics of the main slip patch of the earthquake. Paneldillustrates the case of a very large shallow earthquake, that is, the 23 June 2001 Peru event (Mw=8.4). The variability of the individual STFs (grey lines) does not prevent the extraction of a global behaviour (red line). Figure 2 also illustrates why F m can be more objectively determined than T . Independent information on the temporal earthquake characteristics is provided by the low-frequency wave studies (GCMT [26] , [27] , W Phase [28] ), which determine the centroid time. Abnormally long or short earthquakes induce a shift of the centroid time, which can be used to detect unusual events [29] . However, such approaches mainly allow first-order analyses, as they assume that the STF is an isosceles triangle with fixed duration (in this case, the duration T is twice the centroid time). This hypothesis is not always verified as a number of earthquakes have two or more peaks of seismic moment release (a classical example is the 2007 Pisco (Peru, M w =8.1) earthquake [30] ), or have a long-lasting ‘tail’ after a major peak of moment release. Departures from this assumption can explain part of the dispersion observed between the double of the centroid time and SCARDEC STF duration T (see Supplementary Fig. S4 ). Figure 2: Determining the characteristics of the STFs. In all subfigures, the STFs extracted from P waves recorded at individual seismic stations are shown in light grey and their averages are shown in thick red. The duration T of the average STF is indicated by the black arrow and the peak value F m is shown by the green arrow. The end of the rupture (required to determine T ) is defined here by the last point where the average STF is larger than 0.1 F m . Panels a – c demonstrate three M w =6.6 earthquakes, occurring in Chile (14 July 2010, depth=23 km), Indonesia (11 November 2008, depth=107 km) and Papua New Guinea (11 December 2005, depth=9 km), respectively. These three cases are displayed with the same horizontal and vertical scales to illustrate the differences. The Chile earthquake ( a ) is a classical shallow earthquake, with a simple smooth STF. T and F m are on the order of 9 s and 1.6 10 18 Nm s −1 , respectively. The Indonesia earthquake ( b ) is also simple, but like most deep earthquakes, its duration T (3–4 s) is shorter and its peak value F m (4.7 10 18 Nm s −1 ) is larger. The Papua New Guinea earthquake ( c ) illustrates the case of a more complex STF, where several subevents are present and where the determination of the end of the rupture is dependent on subjective criteria. The total duration T is then more uncertain, and its meaning is more difficult to interpret. On the other hand, F m can still be objectively measured and can be related to the characteristics of the main slip patch of the earthquake. Panel d illustrates the case of a very large shallow earthquake, that is, the 23 June 2001 Peru event ( M w =8.4). The variability of the individual STFs (grey lines) does not prevent the extraction of a global behaviour (red line). Full size image Self-similarity of shallow earthquakes In Fig. 3a,b , F m and T are plotted as a function of seismic moment, with colours scaled to earthquake depth. As expected, in a self-similar model where stress and strain drop depend little on the magnitude, the logarithmic relations tend to show slopes close to two-third and one-third for F m and T , respectively. However, a systematic increase of F m and a systematic decrease of T are observed for deep earthquakes, implying that the product V S Δ σ 1/3 increases with depth. 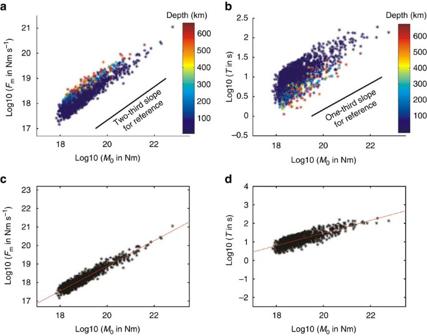Figure 3: Depth and magnitude dependence ofFmandT. (a,b) show the dependence ofFmandT, respectively, as a function of the seismic moment for the global SCARDEC catalogue (about 1,700 earthquakes). The expected tendencies (slope of two-third forFmand one-third forT) in the logarithmic plots are apparent, but the colours (scaled to earthquake depth) reveal a systematic trend: deep earthquakes have a largerFmand a shorterT. When selecting only shallow earthquakes (<50 km;c,d), the linear relationship is clearer; the equations of the best-fit least-squares regression (red lines) arey=0.679x+5.33 andy=0.342x–5.36 forFmandT, respectively. Correlation quality is 0.96 forFmand 0.81 forT. This indicates that shallow earthquakes satisfy the hypothesis that stress (and strain) drop does not vary with magnitude (see main text). Figure 3c,d restricts the analysis to earthquakes shallower than 50 km (~1,200 events), which significantly reduces the variability for a given seismic moment. The best linear fit for peak value F m implies that its seismic moment dependency follows the law = (with α= 10 5.33 and β= 0.679). On the other hand, duration T follows the law = (with γ = 10 −5.36 and δ= 0.342). The exponents are close to the two-third and one-third and have large correlation coefficients, indicating that the stress drop does not depend on the earthquake size for shallow earthquakes in the magnitude range 6< M w <9. Figure 3: Depth and magnitude dependence of F m and T . ( a , b ) show the dependence of F m and T , respectively, as a function of the seismic moment for the global SCARDEC catalogue (about 1,700 earthquakes). The expected tendencies (slope of two-third for F m and one-third for T ) in the logarithmic plots are apparent, but the colours (scaled to earthquake depth) reveal a systematic trend: deep earthquakes have a larger F m and a shorter T . When selecting only shallow earthquakes (<50 km; c , d ), the linear relationship is clearer; the equations of the best-fit least-squares regression (red lines) are y= 0.679 x +5.33 and y= 0.342 x –5.36 for F m and T , respectively. Correlation quality is 0.96 for F m and 0.81 for T . This indicates that shallow earthquakes satisfy the hypothesis that stress (and strain) drop does not vary with magnitude (see main text). Full size image At the global scale, no systematic behaviour is identified inside this shallow depth range, a finding similar to that by Allmann and Shearer [3] . This does not mean that specific trends do not exist for some types of earthquakes. The most documented case is the interplate subduction earthquake class, whose duration has been shown to decrease when moving from the surface to 50 km depth [16] . However, in a global catalogue, this tendency is not apparent because very shallow earthquakes can also have brief durations, for example, in intraplate contexts [3] , [17] . More generally, the differences between individual earthquakes may be significant for a number of reasons (for example, variations of the rupture velocity of the tectonic context; specific properties of the infrequent large strike-slip events, and so on), but they merely add variability to the regression lines in Fig. 3 , without perturbing the main trend. Strain drop invariance To quantify the depth effects, the values, scaled at shallow depth, of the STF peaks ( ) and durations ( = T/ ) are now considered. These individual scaled values and their averages over intervals of depth are shown in Fig. 4 . By construction, the averaged values are very close to one for the shallowest depth interval. The depth dependence is very clear, as almost none of the earthquakes deeper than 100 km has values lower than unity or values larger than unity. Two simple models are potentially able to match the depth evolutions of and . 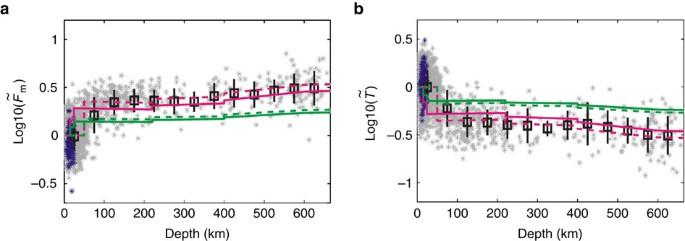Figure 4: STF depth evolution compared with constant strain drop or stress drop models. (a) Depth evolution of, the scaled peak value of the STF. (b) Depth evolution of, the scaled duration of the STF. Stars represent the individual earthquake values and black squares show their averages over depth intervals of 50 km. The s.e. are shown by the vertical thick bars. To show the specific behaviour of shallow subduction interface earthquakes, the 112 offshore thrust events with a dip and depth shallower than 25° and 25 km, respectively, are coloured in blue, whereas all the other earthquakes are shown in grey. Shallow subduction interface earthquakes have anvalue 15% lower than the average of all shallow earthquakes. Coloured green and magenta curves are possible models, calculated with PREM31, considered to explain the observed depth evolution. The solid green and magenta curves correspond to the hypotheses of constant stress drop and constant strain drop, respectively (see main text). The dashed magenta curve corresponds to the constant strain drop model in a modified PREM structure; compared with the original PREM model, the rigidity is lower at shallow depth (VS0equal to 3 km s−1andρ0equal to 2,200 kg m−3) and the transition to upper mantle occurs at 50 km depth. The dashed green curve also takes into account these modifications for the constant stress drop model. Using equations (3) and (4), in a constant stress drop model, we have: Figure 4: STF depth evolution compared with constant strain drop or stress drop models. ( a ) Depth evolution of , the scaled peak value of the STF. ( b ) Depth evolution of , the scaled duration of the STF. Stars represent the individual earthquake values and black squares show their averages over depth intervals of 50 km. The s.e. are shown by the vertical thick bars. To show the specific behaviour of shallow subduction interface earthquakes, the 112 offshore thrust events with a dip and depth shallower than 25° and 25 km, respectively, are coloured in blue, whereas all the other earthquakes are shown in grey. Shallow subduction interface earthquakes have an value 15% lower than the average of all shallow earthquakes. Coloured green and magenta curves are possible models, calculated with PREM [31] , considered to explain the observed depth evolution. The solid green and magenta curves correspond to the hypotheses of constant stress drop and constant strain drop, respectively (see main text). The dashed magenta curve corresponds to the constant strain drop model in a modified PREM structure; compared with the original PREM model, the rigidity is lower at shallow depth ( V S0 equal to 3 km s −1 and ρ 0 equal to 2,200 kg m −3 ) and the transition to upper mantle occurs at 50 km depth. The dashed green curve also takes into account these modifications for the constant stress drop model. Full size image where V S0 is the shear velocity at shallow depth. As the shear velocity increases with depth, this model predicts an increase of and a decrease of . However, as shown by the solid green curves in Fig. 4 , the simple ratio of the shear velocities deduced from the Preliminary Reference Earth Model (PREM) [31] underpredicts the observations. This implies that stress drop increases with depth, by a factor of about 6, between shallow earthquakes and 600-km-deep earthquakes. An alternative model is a constant strain drop model, which means that the stress drop increase with depth is only related to the rigidity increase. In this case, using equations (5) and (6), we predict: where ρ 0 is the density at shallow depth. The depth dependence is now larger and is able to almost reproduce the observations, as indicated by the solid magenta curves in Fig. 4 . In particular, the large contrast between shallow and lithospheric depths (around 100 km) is well reproduced, as is the small and regular tendency inside the upper mantle. The dashed magenta curves in Fig. 4 show that observations can be even closer to the constant strain drop model if ρ 0 and V S0 are lower than the PREM values. This hypothesis appears realistic as the majority of shallow earthquakes occur in damaged zones (for example, along the subduction interfaces), where rigidity is expected to be lower than its global average [16] . We provide in Fig. 4 an observational validation of this hypothesis—consistent with ref. 17 —as shallow subduction interface earthquakes (blue crosses) tend to have a lower (and a longer ) than other shallow earthquakes. If considering the suggested dependence of rupture velocity with depth [5] , [18] by assuming that the average ratio between rupture velocity and shear velocity decreases from 0.8 for shallow earthquakes to 0.6 for 600-km-deep earthquakes, a modest increase of the strain drop with depth is present. As the strain drop variation depends on the cube of the ratio, strain drop should change by a factor of 2.4–3 (and stress drop by a factor of 14–18) when moving from the surface to the deepest seismogenic zones. These observations show that, whatever their magnitude and depth, large earthquakes keep on average a similar ratio between characteristic dimension and average slip over this dimension. A further inspection of the correlation qualities presented in Fig. 3c,d provides insight on the meaning of the word ‘characteristic’. In fact, F m has a larger correlation with seismic moment than T (0.96 and 0.81, respectively) and F m can be related to the dominant slip patch of the earthquake (whereas T is related to the whole earthquake process). The observation that F m follows self-similarity better than T , therefore, indicates that the main slip zone of the earthquakes expands in both directions of the fault plane in a similar manner. The ratio between the average slip and the main patch dimension is independent of the size and depth of the events. The absolute value of this ratio depends on some additional hypotheses (for example, rupture velocity and location of the nucleation point inside the patch), but typical values are in the range 10 −4 –10 −5 . Concretely, the amount of slip on a circular patch with a diameter of 10 km is typically 0.1–1 m. The variability is much more directly determined from the s.e. of F m ( Fig. 4 ), which are equal to ±40% of the mean values. This implies that the strain drop, depending on the cube of F m , can only vary by a factor of 8 at the 95% confidence level. These findings have direct implications when building shallow earthquake scenarios, with the scope of simulating realistic ground motions. Such approaches require us to take into account the sources of uncertainty: one of the main crucial ones concerns the characteristics of the source model [32] . It has been recently shown [33] that the stress drop variability inferred from studies using the corner frequency approach [3] is too large to explain the variability of the observed ground motions. This apparent paradox is explained, to a large extent, by the robust F m estimation of the strain and stress drops, which reduces their variability by a factor of 2. Future studies will aim at further quantifying the relations between source and seismic radiation variability. The stability of the strain drop (both in terms of absolute value and of its limited variability) is also a new constraint on the possible mechanisms of earthquake generation. Shallow earthquakes are thought to originate from the rapid frictional weakening of a fault surface, occurring when shear stress exceeds mechanical friction [34] , [35] . Numerical and laboratory experiments based on this behaviour have been able to mimic the seismic waves generated by earthquakes. However, this rupture process should not operate at depths larger than a few tens of kilometres because of too high a confining pressure. Alternative mechanisms are therefore proposed for deep earthquakes, including dehydration embrittlement, anti-crack faulting in a metastable phase and plastic instability [5] , [6] . Paradoxically, although the physics should be different, most of the seismological observables for deep earthquakes are similar to shallow earthquakes [36] . In particular, deep earthquakes also exhibit a double-couple mechanism, indicating slip on a planar surface. The present study indicates that deep and shallow earthquakes differ little even in key aspects of the rupture process: the strain drop invariance implies that the ratio between seismic slip and rupture dimension remains the same. This finding naturally suggests the hypothesis that a single mechanism, for example, plastic instability [37] , could be responsible for all earthquakes. The existence of several mechanisms, each corresponding to a specific depth range, cannot be ruled out; however, in this case, the difference in their physics should have little repercussion on the resulting earthquake source properties. How to cite this article: Vallée, M. Source time function properties indicate a strain drop independent of earthquake depth and magnitude. Nat. Commun. 4:2606 doi: 10.1038/ncomms3606 (2013).